Dust emission reduction enhanced gas-to-particle conversion of ammonia in the North China Plain Ammonium salt is an important component of particulate matter with aerodynamic diameter less than 2.5 µm (PM 2.5 ) and has significant impacts on air quality, climate, and natural ecosystems. However, a fundamental understanding of the conversion kinetics from ammonia to ammonium in unique environments of high aerosol loading is lacking. Here, we report the uptake coefficient of ammonia (γ NH3 ) on ambient PM 2.5 varying from 2.2 × 10 −4 to 6.0 × 10 −4 in the North China Plain. It is significantly lower than those on the model particles under simple conditions reported in the literature. The probability-weighted γ NH3 increases obviously, which is well explained by the annual decrease in aerosol pH due to the significant decline in alkali and alkali earth metal contents from the emission source of dust. Our results elaborate on the complex interactions between primary emissions and the secondary formation of aerosols and the important role of dust in atmospheric chemistry. Ammonia is the most abundant alkaline gas in the atmosphere, with global emissions estimated to be greater than 58 Tg(N) Yr −1 [1] . Both natural and anthropogenic sources, including soils, oceans, fertilizers, livestock, automobiles, biomass burning, etc., contribute to atmospheric NH 3 [2] , [3] , [4] , [5] . In the atmosphere, NH 3 is responsible for neutralizing sulfuric and nitric acids formed through the oxidation of SO 2 and NO x , leading to the formation of NH 4 + [6] , which is an important component of atmospheric particulate matter (PM) [7] and has significant impacts on air quality, climate, and natural ecosystems [8] , [9] . Atmospheric concentrations of NH 3 vary from several to several tens of ppbv (parts per billion in volume) [10] and show upwards trends over several of the world’s major agricultural regions [11] , [12] , [13] , [14] . NH 3 emissions in China were estimated to be ~10 Tg in the 2000s [9] , [15] , [16] and exceeded the sum of those in the European Union and the United States [9] . Modeling studies revealed that NH 3 is an essential controlling factor regarding sulfate (SO 4 2− )-nitrate (NO 3 – )-ammonium (SNA) aerosol and fine particle pollution over China [9] , [17] . The relative contribution of ammonium nitrate to PM 2.5 (with an aerodynamic diameter of PM less than 2.5 μm) increases as a function of PM mass concentrations at urban sites [18] , [19] . The concentrations of NO 3 – and NH 4 + in Beijing increased at rates of 0.8 and 0.6 μg m −3 Yr −1 , respectively, as the concentration of SO 4 2− decreased obviously after 2013 [17] , [20] . Furthermore, ammonia is important for atmospheric new particle formation (NPF) in megacities [21] . Therefore, it is very important to understand the conversion kinetics from NH 3 to NH 4 + in the atmosphere. Thermodynamic models assume that NH 3 uptake and particle neutralization occur within a model time step (usually from several seconds to minutes), as inferred from laboratory studies [22] , [23] . The NH 3 uptake kinetics will thus significantly affect the ability of models to properly predict the transport of NH 3 and NH 4 + [23] , [24] , [25] , [26] . The uptake kinetics of NH 3 on aerosol particles are scarce, although a few studies have reported the uptake coefficient (γ NH3 ) or accommodation coefficient (α) of NH 3 on model particles such as ice [27] , sulfuric acid/H 2 O [22] , [28] , [29] , [30] , [31] , [32] , organic acids [28] , [33] and organic aerosols (OA) [34] , with the γ NH3 values varying from 10 −4 to 1.0. In the atmosphere, numerous air pollutants have a complicated influence on the uptake kinetics of trace gases, including NH 3 . Liggio et al. [23] reported that the γ NH3 on sulfuric acid aerosols varied from 4 × 10 −3 to 2 × 10 −4 when the OA-to-sulfate mass ratio was from 0.14 to 0.55, in contrast to ~1.0 for the organic-free system. Similar retardancy effects were also observed for the uptake of NH 3 by sulfuric acid aerosols precoated with n -hexadecanol [35] and n -hexadecane [36] . The composition and mixing state of atmospheric PM should be more sophisticated than those simulated in the laboratory. However, the uptake coefficient of NH 3 on real ambient PM is currently lacking. It is also unknown how the conversion kinetics changes in the atmosphere. In this article, we demonstrate the γ NH3 on ambient PM 2.5 in the North China Plain (NCP) based on long-term field observations. We show that the γ NH3 on ambient PM 2.5 is significantly lower than those on model aerosol particles, while it increases annually in the statistical sense driven by an increase in aerosol acidity. By comprehensively analyzing the chemical composition and source apportionment of aerosol particles, we find that the reduction of alkali and alkali earth metals from dust emissions resulted in an increase in aerosol acidity, although the ratio of sulfate-to-nitrate in PM 2.5 slightly decreases, followed by the conversion kinetics from NH 3 to NH 4 + . The overall goal of this work is to provide a fundamental understanding of particle-phase NH 4 + formation in the context of decreasing the mass loading of sulfate in aerosol particles. Variations in NH 4 + and NH 3 As shown in Fig. 1 , the mass concentrations of NH 4 + and non-NH 4 + water-soluble ions in Shijiazhuang are 0.052–89.0 μg m −3 (median value of 7.5 μg m −3 ) and 0.9–241.2 μg m −3 (median value of 22.6 μg m −3 ), respectively, during the observation period (from March 15, 2018 to November 15, 2020). The corresponding values in Beijing are 0.06–47.7 μg m −3 (median value of 3.5 μg m −3 for NH 4 + ) and 0.07–212.5 μg m −3 (median value of 9.1 μg m −3 for non-NH 4 + ions). Compared with the previous observations, the air quality in both Shijiazhuang and Beijing has been significantly improved. For example, the mean concentration ±σ (standard deviation) of water-soluble NH 4 + (10.5 ± 10.2 μg m −3 ) in Shijiazhuang is significantly lower than that (13.8 ± 13.6 μg m −3 ) measured from June 2014 to April 2016 [37] . In Beijing, it is also lower (5.5 ± 5.6 μg m −3 ) than that measured from February to November 2017 [38] and even lower than the NH 4 + concentration in nonrefractory PM 1 (8.5 ± 7.9 μg m −3 ) from July 2011 to June 2012 [39] . Fig. 1: Concentrations of particulate NH 4 + , non-NH 4 + ions and gas-phase NH 3 . The time series of ( a , b ) mass concentrations of particulate NH 4 + and non-NH 4 + in water-soluble ions, ( c , d ) the relative fraction of particulate NH 4 + and non-NH 4 + ions, and ( e , f ) gas-phase NH 3 in Shijiazhuang (SJZ) and Beijing (BJ). Full size image The concentration of gas-phase NH 3 in Shijiazhuang varies from 0.02 to 89.5 μg m −3 with a median value of 22.1 μg m −3 , while it is from 1.0 to 43.2 μg m −3 with a median value of 15.6 μg m −3 in Beijing. The median value of NH 3 concentrations in Beijing is comparable with previous observations carried out in Beijing and Xi’an [40] but higher than that in Shanghai (4.6 μg m −3 ) [2] . It should be noted that the concentration of gas-phase NH 3 shows a weak downwards trend in Shijiazhuang from March 2018 to November 2020 (Fig. 1e ). The decreasing rate ±σ of NH 3 is 2.3 ± 0.1 µg m −3 Yr −1 according to linear fitting. This value is almost the same as the decreasing rate (2.3 ± 0.4 µg m −3 Yr −1 ) fitted according to a combination of a sine function (due to seasonal variations of NH 3 emissions [2] , [41] and partition [42] ) and a linear function (due to annual changes of NH 3 emissions) for the probability-weighted NH 3 concentrations based on a 2D Kernel density plot (Supplementary Fig. 1 ) by binning the dataset into 100×100 boxes to decrease the signal noise [43] . As shown in Fig. 1c , however, the relative fraction of NH 4 + in water-soluble ions is stable annually in Shijiazhuang. We even observe a slight upwards trend for the fraction of NH 4 + in inorganic anions or nonrefractory PM 2.5 measured by a Time-of-Flight Aerosol Chemical Speciation Monitor (ToF-ACSM, Aerodyne) in Beijing (Supplementary Fig. 2 ). This is in agreement with previous results that the NH 4 + fractions increased significantly in Beijing from 2014 to 2019 [44] . These results strongly imply that the partition equilibrium between gas-phase NH 3 and particle-phase NH 4 + interannually prefers particle-phase NH 4 + in both Shijiazhuang and Beijing. Kinetics We calculate the nocturnal γ NH3 to decrease the influence of nucleation through gas-phase H 2 SO 4 or HNO 3 and NH 3 as well as variations of advection and deposition on the γ NH3 calculations (the details can be seen in the SI). In Shijiazhuang, the derived nocturnal γ NH3 values are in the range of 4.02 × 10 −8 to 8.02 × 10 −2 with mean ±σ and median values of (1.13 ± 12.4) × 10 −4 and 6.37 × 10 −5 (Fig. 2 ), respectively. Although a variation in γ NH3 is discernible, no significant difference among different seasons is observed at the 0.05 level due to the noisy data, with mean ±σ γ NH3 values of (2.22 ± 6.87) × 10 −4 , (2.21 ± 4.20) × 10 −4 , (2.88 ± 7.70) × 10 −4 and (2.52 ± 21.6) × 10 −4 in spring, summer, autumn and winter, respectively, in Shijiazhuang (Supplementary Fig. 3 ). The γ NH3 values, which vary from 1.24 × 10 −6 to 9.70 × 10 −2 in Beijing, are comparable to those in Shijiazhuang during the same observation periods (Fig. 2a ). The mean γ NH3 values reported here are significantly smaller than the γ NH3 on sulfuric acid (0.1–1) [29] , [30] , [32] , aqueous surfaces (~5 × 10 −3 –0.1) from pH in the range of 0–13 [31] and acidified secondary organic aerosol (~10 −3 –~10 −2 ) [34] , while they are comparable with those on the surface of ice (5.3 ± 2.2 × 10 −4 ) [27] and sulfuric acid in the presence of organic gases (2 × 10 −4 –4 × 10 −3 ) [23] . Fig. 2: The variations of nocturnal uptake coefficient of NH 3 (γ NH3 ). a Time series of nocturnal γ NH3 in Shijiazhuang (SJZ) and Beijing (BJ), b probability distribution of nocturnal γ NH3 in Shijiazhuang, and c probability-weighted nocturnal γ NH3 in Shijiazhuang and Beijing. The equation of the dashed line is γ NH3 = 2.50 × 10 −4 + 6.58 × 10 −5 t ( R = 0.83, t : year). Full size image γ NH3 shows an obvious upwards trend but with obvious variations in Fig. 2a . Figure 2b shows the probability distribution of nocturnal γ NH3 in Shijiazhuang, and Fig. 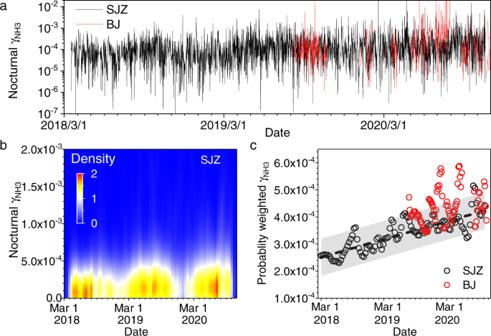Fig. 2: The variations of nocturnal uptake coefficient of NH3(γNH3). aTime series of nocturnal γNH3in Shijiazhuang (SJZ) and Beijing (BJ),bprobability distribution of nocturnal γNH3in Shijiazhuang, andcprobability-weighted nocturnal γNH3in Shijiazhuang and Beijing. The equation of the dashed line is γNH3= 2.50 × 10−4+ 6.58 × 10−5t(R= 0.83,t: year). 2c shows the probability-weighted nocturnal γ NH3 after the time series of γ NH3 is converted into a 2D kernel density plot. Three peaks with a high frequency of large γ NH3 occur in summer, while two minima are present in winter. The probability-weighted γ NH3 , which statistically indicating weighted mean γ NH3 , shows obvious seasonal variations and interannually increases with relative time in Shijiazhuang, e.g., γ NH3 = 2.50 × 10 −4 + 6.58 × 10 −5 t ( R = 0.83, t : year) or γ NH3 = 2.47 × 10 −4 –6.0 × 10 −5 sin(π( t + 1.99)/0.55) + 6.99 × 10 −5 t ( R = 0.35, t : year). The probability-weighted γ NH3 values in Beijing are slightly higher than those in Shijiazhuang during the same period. They are more scattered due to the small dataset in Beijing than that in Shijiazhuang. However, a weak upwards trend is still observable in Beijing (Fig. 2c , R = 0.40) with a comparable slope of 5.15 × 10 −5 Yr −1 . These results mean that the γ NH3 increase by 6.24 ± 0.97 × 10 −5 per year in the NCP, which further confirms the assumption that the formation of particle-phase NH 4 + is preferred recently from the point of view of conversion kinetics. Driving force for the enhancement of γ NH3 A chemical reaction is usually sensitive to temperature. A low activation energy of 12.5 kJ mol −1 has been reported for the reaction between H 2 SO 4 and NH 3 [30] . However, the decomposition of ammonium is more sensitive to temperature than the forward reaction [42] . Thus, a negative temperature dependence has been observed for the uptake of NH 3 on the surface [31] , [42] . This means that the high temperature in summer should be unfavorable for the uptake of NH 3 in the atmosphere. The formation of NH 4 + includes the uptake of NH 3 and the proton transfer reaction between protons (H + ) and NH 3 . The positive dependence of γ NH3 on acidity for the uptake of NH 3 on aqueous surfaces [31] or organic aerosol surfaces [34] has been reported previously. As shown in Fig. 3a, b , the aerosol pH values, which dominantly varies from 3.0 to 7.0 calculated using the ISORROPIA II model in Beijing and Shijiazhuang, are overall higher than those estimated in Nagoya, Japan (3.6–5.4) [45] , the cities in the Po Valley, Italy (1.5−4.5) [46] , and the northeastern United States (0.5–3) [47] , while they are comparable with those reported in northern China [44] , [48] , [49] , [50] , [51] . The relatively high aerosol pH in the NCP can be explained by the high concentrations of NH 3 and dust in the atmosphere to neutralize sulfate and nitrate [52] . Fig. 3: The aerosol pH and its correlation with nocturnal uptake coefficient of NH 3 (γ NH3 ). a The probability distribution of the nocturnal aerosol pH in Shijiazhuang (SJZ), b the probability-weighted nocturnal aerosol pH in Shijiazhuang and Beijing (BJ), c , d the relationship between the nocturnal γ NH3 and the aerosol pH in Shijiazhuang and Beijing. Full size image Seasonal variations in aerosol pH are obvious (Fig. 3a, b ), e.g., high aerosol pH in winter and low aerosol pH in summer. This is determined in a complicated manner by the composition of PM 2.5 , the air temperature, and the aerosol liquid water content (AWC) or RH [45] , [46] , [48] , [50] , [53] . The probability-weighted aerosol pH can be well fitted by a combination of a sine function which reflects the seasonal variation of aerosol pH, inversely depending on temperature [54] and the ratio of SO 4 2− /NO 3 − [46] , and a linear function of time that reflecting interannual changes of aerosol pH, i.e., pH = 4.90–1.06sin(π( t − 0.58)/0.51) – 0.18 t ( R = 0.88, t : year) in Shijiazhuang and pH = 4.98–0.81 sin(π( t − 0.80)/0.44)–0.27 t ( R = 0.69, t : year) in Beijing. This means that the aerosol acidity ±σ increases by 0.23 ± 0.06 units per year. This is consistent with the interannual increase in γ NH3 (Fig. 2b ). It should be noted that Song et al. [44] observed a decrease in wintertime aerosol acidity from 2014 to 2019. In their work, the aerosol pH values were modeled using gaseous ammonia and chemical components of nonrefractory submicron particles (NR-PM 1 ), including SO 4 2− , NO 3 − , NH 4 +, and Cl − , as inputs. In this study, however, more inputs, including the measured gas-phase (NH 3 , HCl, and HNO 3 ) and particle-phase (SO 4 2− , NO 3 − , Cl − , NH 4 + , K + , Na + , Ca 2+, and Mg 2+ ) components, are accounted for. This should result in a more precise aerosol pH. Figure 3c, d further show the relationship between γ NH3 and aerosol pH. 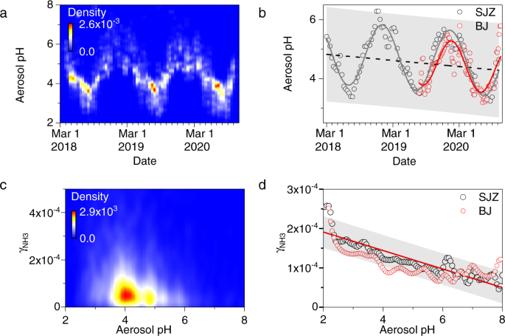Fig. 3: The aerosol pH and its correlation with nocturnal uptake coefficient of NH3(γNH3). aThe probability distribution of the nocturnal aerosol pH in Shijiazhuang (SJZ),bthe probability-weighted nocturnal aerosol pH in Shijiazhuang and Beijing (BJ),c,dthe relationship between the nocturnal γNH3and the aerosol pH in Shijiazhuang and Beijing. The probability-weighted γ NH3 and aerosol pH show a linear correlation, i.e., γ NH3 = 2.38 × 10 −4 –2.35 × 10 −5 pH ( R = 0.90, in Shijiazhuang) and γ NH3 = 2.06 × 10 −4 –1.90 × 10 −5 pH ( R = 0.63, in Beijing). This is consistent with the positive correlation between the k het of NH 3 and the acidity of aerosols, expressed by the H + /NH 4 + mole ratio [55] . The negative correlation between γ NH3 and aerosol pH can be well explained in light of the linear free energy relationship for a reaction series [56] , which is also observed in our previous work on the uptake of amines by ammonium salts [57] and organic acids [58] . In addition, these results are in agreement with the formation of NH 4 NO 3, which is HNO 3 sensitive according to the partition of nitric acid and ammonia to the aerosol phase [59] (Supplementary Fig. 4 ). Silvern et al. [34] found that aerosols are becoming more acidic even as SO 2 emissions decrease and ammonia emissions remain constant in the United States. They proposed that sulfate particles are increasingly coated by organic matter (OM), retarding the uptake of ammonia similar to that observed in chamber studies [23] . However, we do not observe an increase in the OM/sulfate ratio during our observations, as shown in Supplementary Fig. 5 . In addition, the OM/sulfate ratios in Beijing are higher than those in Shijiazhuang, while both the aerosol pH and the γ NH3 are comparable in these two locations. Recent studies proposed that conversion process from NOx to NO 3 − could affect the conversion process from NH 3 to NH 4 + [60] . Although a seasonal variation of the NOR is observable, i.e., higher NOR values are observed in winter compared to summer, the probability-weighted nitrogen oxidation ratio (NOR) is annually stable during our observations in Shijiazhuang (Supplementary Fig. 6 ), unlike the observed γ NH3 or pH. These results mean that the annual increase in aerosol pH should not be mainly regulated by the organic film in aerosols since inorganic and organic compounds are expected to reside in separate phases in Beijing [44] or variations in NOR. The composition should be the important factor affecting the annual increase in aerosol acidity [45] , [46] , [47] , [53] because we do not observe interannual variations in AWC and temperature (Supplementary Fig. 7 ). SO 4 2− , NO 3 − , NH 4 + , and other cations (K + , Na + , Ca 2+ , Mg 2+ ) are the major components that influence the aerosol pH. Figure 4 shows the monthly mean ratios of NH 4 + /other cations, SO 4 2− /NO 3 − as well as the corresponding mass concentrations. 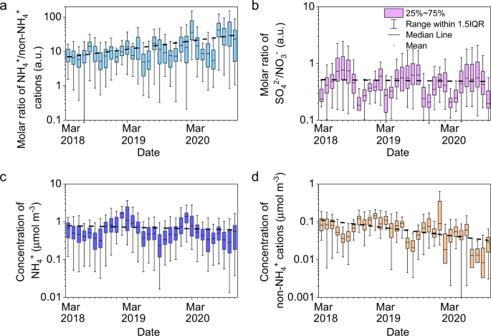Fig. 4: The variations of NH4+, non-NH4+cations, SO42−and NO3−. a,bThe monthly mean values of the ratios of NH4+/other cations and SO42−/NO3−;c,bthe mass concentrations of NH4+and other cations in Shijiazhuang. The dashed lines are a linear fit of the monthly mean values. 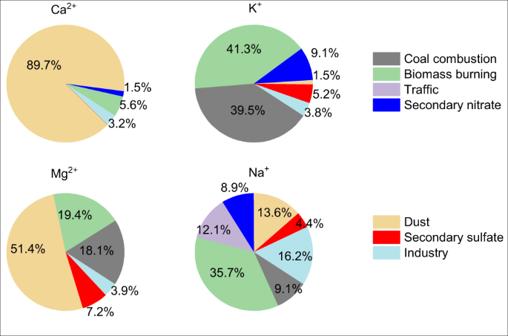Fig. 5: The sources of soluble alkali metals in PM2.5. The relative mean contribution from coal combustion, biomass burning, traffic, secondary nitrate, dust, secondary sulfate and industry sources to the mass concentrations of Ca2+, Mg2+, K+and Na+ions. The ratio of SO 4 2− /NO 3 − shows a weak decreasing trend. This should not result in the interannual enhancement of aerosol acidity because it is positively correlated with the ratio of SO 4 2− /NO 3 − [46] . In contrast, an upwards trend for the ratio of NH 4 + /other cations is observable in Fig. 4a . Additionally, NH 4 + shows a weak down or relatively stable trend, while a more obvious reduction of other cations can be seen in Fig. 4d . Ca 2+ contributes 55.1 ± 20.3% to the total mass of these alkali and alkali earth metals. It is well known that the basicity of NH 4 + is significantly weaker than that of alkali and alkali earth metals. In addition, Ca 2+ can react with SO 4 2− to form insoluble CaSO 4 , which is out of the aerosol aqueous phase, subsequently reducing the aqueous SO 4 2− and thus the particle acidity [61] . The decrease in Ca 2+ concentration thus inevitably leads to a weakened neutralization or precipitation ability to acids. In previous work, it has also been found that mineral dust plays an important role in decreasing aerosol pH [53] , [61] , [62] , [63] . These results strongly imply that the interannual reduction in aerosol pH should be dominated by the decline in alkali and alkali earth metals [64] in both Shijiazhuang and Beijing. Fig. 4: The variations of NH 4 + , non-NH 4 + cations, SO 4 2− and NO 3 − . a , b The monthly mean values of the ratios of NH 4 + /other cations and SO 4 2− /NO 3 − ; c , b the mass concentrations of NH 4 + and other cations in Shijiazhuang. The dashed lines are a linear fit of the monthly mean values. Full size image To further confirm the importance of alkali and alkali earth metals to aerosol pH, machine learning has been performed using a random forest model [65] , which is a highly accurate classification algorithm. Twenty-three meteorological and chemical parameters are used as inputs to investigate their effect on aerosol pH. Ca 2+ is the third most important factor after temperature and RH to aerosol pH (Supplementary Fig. 8 ). Mg 2+ , K + , and Na + also significantly contribute to aerosol pH. These results are consistent with the decreased fugitive dust emissions in the North China Plain due to the intensive regulation of dust emissions [66] , [67] , [68] . It should be pointed out that organics are not considered when we calculate aerosol pH. If the fraction of organic acids increases annually during our observations, it should also lead to an upwards trend in aerosol acidity. The mass fraction of m/z 44 ( f 44 ), which is usually an indicator of carboxylic acids in OA [69] , is interannually stable, although f 44 varied seasonally in Beijing (Supplementary Fig. 9 ). Therefore, we can conclude that the interannually elevated aerosol acidity should not be determined by the variations in organic acid content although aerosol acidity might be underestimated by the ISORROPIA II model that cannot consider organic acids. Seven sources of PM 2.5 , including coal combustion, biomass burning, traffic, secondary nitrate, dust, secondary sulfate, and industry, have been identified in Shijiazhuang using the measured concentrations of inorganic ions, OC, EC, and heavy metals. The Q true /Q exp is 4.3 for the seven-factors solution. This value corresponds to a relatively stable variation of the d(Q true /Q exp )/dN (Supplementary Fig. 10 ). Supplementary Figs. 11 and 12 show their source profiles and the time series of hourly mean mass concentrations. Coal combustion is characterized by high loadings of OC, EC, and heavy metals; biomass burning is characterized by high concentrations of Cl and K and moderate OC and EC; traffic shows a high fraction of Zn and moderate concentrations of EC and OC; dust sources show high fractions and concentrations of Ca 2+ , Mg 2+ , Al and Ti; secondary nitrate and secondary sulfate are characterized by high concentrations of nitrate and sulfate, respectively; industrial sources are connected with high concentrations of Fe, Co, Mn, etc. These sources are well supported by the diurnal and monthly variations (Supplementary Fig. 13 ). The mean ± σ contributions of these 7 sources to the PM 2.5 mass concentration during the observations in Shijiazhuang are 15.3 ± 7.2, 10.6 ± 12.5, 14.6 ± 8.1, 12.3 ± 10.1, 16.9 ± 15.5, 14.6 ± 10.0, and 15.6 ± 11.9%, respectively. As shown in Fig. 5 , dust explains 89.7, 51.4, and 13.6% of the soluble Ca 2+ , Mg 2+ , and Na + , respectively. In addition, the mass concentration of dust decreased obviously (Supplementary Fig. 12 ), with an annual decrease rate of 0.90 ± 0.03 µg m −3 yr −1 . The contribution of dust to PM 2.5 mass concentration also shows a prominent decrease (10.8 ± 2.5% yr −1 ) as shown in Supplementary Fig. 14 . This means that the reduction in dust emissions mainly regulates the increase in aerosol acidity observed in Fig. 3 . Fig. 5: The sources of soluble alkali metals in PM 2.5 . The relative mean contribution from coal combustion, biomass burning, traffic, secondary nitrate, dust, secondary sulfate and industry sources to the mass concentrations of Ca 2+ , Mg 2+ , K + and Na + ions. Full size image Liggio et al. [23] found that competition for uptake between NH 3 and organic gases can block the surface of sulfuric acid aerosols from incoming NH 3 , subsequently slowing the approach to thermodynamic equilibrium. This was further validated by modeling studies that explained the low ammonium-sulfate ratio (1.04 ± 0.21 mol mol −1 ) in the eastern United States, even though ammonia was in large excess [70] . The uptake of NH 3 by sulfuric acid aerosols can also be retarded by precoated n -hexadecanol [35] and n -hexadecane [36] . However, as shown in Supplementary Fig. 5 , the OM/sulfate ratio is relatively stable during our observations. In addition, the OM/sulfate ratio in Beijing is obviously higher than that in Shijiazhuang during the same observational period, while the γ NH3 is comparable between these two locations. This means that the observed interannually increase in γ NH3 cannot be explained by the changes in organic coating. In the atmosphere, the mixing state of aerosols is more complicated than that of model aerosols [71] and subsequently has a complex influence on the reaction kinetics of trace gases, similar to other reaction systems [72] , [73] . Thus, we ascribe the relatively small γ NH3 in this work to the matrix effect of ambient aerosols. On the other hand, Kuwata and Martin [74] showed that the amount and rate of ammonia uptake by secondary organic aerosol depends strongly on RH due to both thermodynamics and the influence of particle viscosity on uptake kinetics. We also observe an obvious increase of the probability-weighted γ NH3 at high RH values, in particular, over 80% of RH (Supplementary Fig. 15 ). However, the interannual changes of RH is not observed. This means that variations of RH might partially contribute to the wide range of the γ NH3 (Fig. 2a ), while it cannot statistically explain the interannual increase of the γ NH3 . It should be noted that the probability-weighted γ NH3 varies from 2.31 × 10 −4 to 5.87 × 10 −4 in the NCP (Fig. 2c ). It is smaller than the measured γ NH3 on model particles, but close to that (5 × 10 −4 ) utilized in a modeling study [70] . Further studies are required for understanding the impacts of γ NH3 values on atmospheric chemistry including nitrogen cycle and PM 2.5 mass loading in the future. NH 3 is mainly neutralized by H 2 SO 4 and HNO 3 . In the daytime, the gas-phase concentration of H 2 SO 4 is estimated to be from 6.35 × 10 5 to 5.49 × 10 6 molecules cm −3 based on a proxy method [75] in Shijiazhuang. The condensed H 2 SO 4 only contributes (0.14 ± 0.17)% to particle-phase NH 4 + and (0.70 ± 1.91)% to particle-phase SO 4 2− . The mean ±σ γ NH3 will be underestimated by (2.0 ± 6.4)% if the condensation of H 2 SO 4 is not accounted for (Supplementary Fig. 16 ). At night, the contribution of gas-phase H 2 SO 4 can be ruled out because it is mainly produced from photochemical oxidation of SO 2 in the daytime, and its nighttime concentration is very low [75] . However, gas-phase HNO 3 might be released through the hydrolysis of heterogeneous hydrolysis of N 2 O 5 at night [76] , [77] , [78] . Although nucleation between HNO 3 and NH 3 at low temperatures and high nitric acid concentrations has been observed in chamber studies [79] , this process has not yet been validated in any field measurements. According to the chamber results, particle growth via nucleation between HNO 3 and NH 3 is active when the product of HNO 3 and NH 3 concentrations ( c HNO3× c NH3 ) is higher than 5 × 10 5 pptv 2 and the temperature is lower than 278.15 K [79] . We have checked the nocturnal dataset with PM 2.5 concentrations lower than 35 μg m −3 and a duration longer than 3 h during our observations. Forty-two events have been picked out with c HNO3× c NH3 larger than 5 × 10 5 pptv 2 ( c HNO3 ± σ: 0.19 ± 0.09 ppbv; c NH3 ± σ: 14.1 ± 10.5 ppbv). However, we do not observe any nucleation or growth event based on the particle size spectrum even though the PM 2.5 mass concentration (20.2 ± 8.9 μg m −3 ) and the temperature (273.6 ± 3.1 K) are low enough. Therefore, we postulate that the contribution of nucleation between HNO 3 and NH 3 to particle-phase NH 4 + should be negligible. It should be noted that the concentrations of ions vary from 3.2 to 30.7 mol L −1, and the ionic strength in the aerosol liquid phase vary from 1.8 to 23.2 mol L −1 during our observations (Supplementary Fig. 17a ). The ISORROPIA II model thus usually overestimates aerosol acidity because it assumes a unity of activity coefficient (γ H+ ) [80] . We have calculated the activity coefficient, which is significantly lower than unity (Supplementary Fig. 17a ), according to the method derived by Glueckauf for concentrated electrolyte solutions [81] , [82] . As shown in Supplementary Fig. 17b , the aerosol pH F (γ H+ = 1.0) values are well correlated with the aerosol pH γ values (slope = 1.09, R = 0.99), which accounted for the γ H+ . However, the aerosol pH F values are lower at 1.27 units (the intercept) than the aerosol pH γ values. This is in agreement with a recent study that found that the pH F calculated by ISORROPIA II was ~1 unit lower than the pH γ calculated by models in which the activity coefficient was accounted for [80] . However, as shown in Supplementary Fig. 17c, d , the pH γ shows similar seasonal and interannual variations as the pH F . This means that the dependence of γ NH3 and aerosol pH (Fig. 3d ) should not be affected by the uncertainty of pH from the activity coefficient of H + . This does so for the relationship between aerosol pH and the content of alkali and alkali earth elements (Fig. 4 ). SO 2 emissions have decreased significantly in Asia since 2005, while NOx emissions show a lower decline rate [83] . This leads to a decrease in the ratio of SO 4 2− /NO 3 − in PM 2.5 [20] , [84] , as observed in the United States [85] . It is well recognized that the concentration of SO 4 2− [45] , [64] , [86] or the ratio of SO 4 2− /NO 3 − [87] can significantly regulate aerosol acidity, i.e., a higher SO 4 2− /NO 3 − traditionally corresponds to a stronger aerosol acidity [45] . Thus, a decrease in aerosol acidity is expected in many regions, including East Asia, because of the shifting inorganic aerosol composition from ammonium sulfate to ammonium nitrate [85] . However, an increase in aerosol acidity is observed in the typical cities of the NCP (Shijiazhuang and Beijing) in this work, although the ratio of SO 4 2− /NO 3 − decreases slightly. A machine learning study and source apportionment have confirmed that a significant reduction in alkali and alkali earth metals compensates for the increase in aerosol pH resulting from the decreased sulfate content in PM 2.5 . The increased aerosol pH favors the uptake of NH 3 in both Shijiazhuang and Beijing, thus leading to a constant or slightly increased NH 4 + fraction in PM 2.5, as observed in this work. NH 4 + can further affect aerosol acidity via both neutralizing [80] , [88] and buffering effects [50] , [85] . Aerosol acidity plays an important role in not only secondary organic aerosol formation, as also recognized in previous studies [89] but also secondary inorganic aerosol formation, as observed in this study, and subsequently aerosol mass loadings and chemical composition. Besides ammonium formation, the formation of sulfate and nitrate is also sensitive to aerosol pH, e.g., a high aerosol pH is in favor of heterogeneous conversion from SO 2 to sulfate [90] , [91] , the partition of semi-volatile nitrate [59] , [63] , and uptake of N 2 O 5 to form nitrate [92] . In addition, strong aerosol acidity favors the dissolution of toxic heavy metals [93] and thus the toxicity of aerosols. In developing regions, the regulation of dust emissions is one of the most effective administration strategies targeting PM 2.5 pollution. Our results mean that more attention should be given to the indirect effects of these strategies on air quality and human health in the future. Field observations Observations were carried out at Aerosol and Haze Laboratory, Beijing University of Chemical Technology (AHL/BUCT Station, Lat. 39°56ʹ31ʺ and Lon. 116°17ʹ52ʺ) from August 8, 2019, to November 15, 2020, and Hebei Atmospheric Supersite, which is in Shijiazhuang University (HAS/SJZ, Lat. 38.0281°, and Lon. 114.6070°) from March 15, 2018, to November 15, 2020. 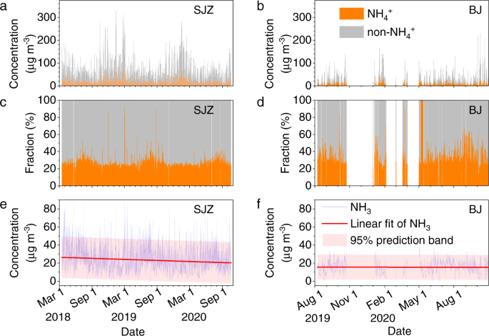The details about the observation stations have been described in previous work [94] , [95] , [96] . Briefly, both were on the rooftop of the corresponding main teaching building (5 floors, ~18 m, and ~23 m, respectively, above the surface for AHL/BUCT and HAS/SJZ stations) and are typical urban observation stations surrounded by traffic and residential emissions. The locations of the stations are shown in Supplementary Fig. 18 . Fig. 1: Concentrations of particulate NH4+, non-NH4+ions and gas-phase NH3. The time series of (a,b) mass concentrations of particulate NH4+and non-NH4+in water-soluble ions, (c,d) the relative fraction of particulate NH4+and non-NH4+ions, and (e,f) gas-phase NH3in Shijiazhuang (SJZ) and Beijing (BJ). The instruments in this study are shown in Supplementary Table 1 . Briefly, the mass concentrations of PM 2.5 were measured using a Taper Element Oscillating Microbalance (TEOM 1405-DF, ThermoFisher) at the AHL/BUCT station and a Beta Attenuation Mass Monitor (BAM-1020, Met One Instruments) at the HAS/SJZ station. Water-soluble ions (Cl − , NO 3 − , SO 4 2− , Na + , NH 4 + , K + , Mg 2+ , and Ca 2+ ) in PM 2.5 and gas pollutants (HCl, HONO, HNO 3 , SO 2, and NH 3 ) were measured using an analyzer for Monitoring AeRrosols and Gases in ambient Air (MARGA, 2060R at the AHL/BUCT station and 2080 at the HAS/SJZ station, Metronhm Process Analytics) with 1 h of time resolution. Trace gases, including NO x , SO 2 , CO, and O 3, were measured with the corresponding analyzer (Thermo Scientific, 42i, 43i, 48i, and 49i). A Particle Size Magnifier (PSM, Airmodus), a Neutral cluster & Air Ion Specter (NAIS, Airel Ltd), a Differential Mobility Particle Sizer (DMPS, Custom made, University of Helsinki), and an Aerodynamic Particle Sizer (APS 3321, TSI) were deployed to measure the particle size distribution from 1 nm to 10 μm at the AHL/BUCT station, while a Scanning Mobility Particle Sizer (SMPS, TSI) consisting of a Differential Mobility Analyzer (DMA 3938, TSI) and a Condensation Particle Counter (CPC 3776, TSI) and an APS (3321, TSI) were available at the HAS/SJZ station. The bulk composition, including chloride, nitrate, sulfate, ammonium, and organics of nonrefractory PM 2.5 (NR-PM 2.5 ), was measured with a time-of-flight aerosol chemical speciation monitor (ToF-ACSM, Aerodyne) at the AHL/BUCT station. Organic carbon (OC) and element carbon (EC) were measured using the National Institute for Occupational Safety and Health (NIOSH, 5409) protocol by OC/EC analyzers (Model 4, Sunset) at both stations. The concentrations of heavy metals were measured using an X-ray fluorescence Atmospheric Heavy Metal Online Analyzer (EHM-X100, Skyray Instruments). Meteorological parameters, including temperature, pressure, relative humidity (RH), wind speed, and direction, were measured using weather stations (ASW310 at the AHL/BUCT station and WXT 520 at the HAS/SJZ station, Vaisala). The MARGAs were externally calibrated using anionic solutions (Cl − , Br − , NO 3 − , SO 4 2− ) and cationic solutions (Li + , Na + , K + , Mg 2+, and Ca 2+ ) monthly. Internal calibration was also carried out hourly using LiBr standard solutions. The detection limits of Cl − , NO 3 − , SO 4 2− , Na + , NH 4 + , K + , Mg 2+ , and Ca 2+ were 0.01, 0.05, 0.04, 0.05, 0.05, 0.09, 0.06 and 0.09 μg m −3 , respectively. All the instruments for trace gas measurements were calibrated weekly using the corresponding standard gases. The detection limits were 0.05, 0.05, 40, and 0.5 ppbv for NO x , SO 2 , CO, and O 3 , respectively. External calibration was performed for the OC/EC analyzers biweekly using sucrose solutions. The heavy metal analyzer was calibrated with external standards. Calculations of γ NH3 and aerosol pH NH 3 mainly reacts with H 2 SO 4 and HNO 3 in the atmosphere. The reaction is a prototypical acid-base neutralization, i.e., proton transfer reaction, which occurs instantaneously in aqueous solutions. Although nucleation through H 2 SO 4 and NH 3 contributes to new particle formation [97] , this process usually cannot explain the high nucleation rates observed in different environments [98] , [99] and the growth of ammonium salts. Nucleation through HNO 3 and NH 3 in the gas phase has not yet been validated in ambient air [70] , although it has been observed in a laboratory study at low temperature and high HNO 3 or NH 3 concentrations [79] . These results mean that NH 3 should mainly contribute to particle growth via heterogeneous uptake. Therefore, the rate constant for conversion from NH 3 to NH 4 + through a heterogeneous reaction can be derived in the same way as calculating the conversion rate constant of NO 2 to HONO [96] , [100] , [101] . As shown in Eq. ( 1 ), 
    k_het=2(c_NH_4^+,t_2-c_NH_4^+,t_1)/(c_NH_3,t_2+c_NH_3,t_1)(t_2-t_1)
 (1) where k het is the quasi-first-order reaction rate constant for heterogeneous conversion (s −1 ) and c NH4+,ti and c NH3 , ti are the concentrations of the particle-phase concentrations of NH 4 + and NH 3 at a given time t i (ppbv or μg m −3 ). The k het was calculated when c NH4+ increases, while c NH3 decreases assuming a constant emission rate from t 1 to t 2 (within 1 h). The nocturnal k het values are 1.3 ± 2.1 × 10 −5 s −1 and 1.2 ± 2.4 × 10 −5 s −1 , respectively, in Shijiazhuang and Beijing. They are in the range of the k het (4.0 × 10 −6 s −1 –4.1 × 10 −4 ) by measuring the conversion of NH 3 to NH 4 + as the air mass traveled between three successive distant sampling points in rural England [55] . Then, the nighttime uptake coefficient of NH 3 (γ NH3 ) was calculated according to 
    γ_NH_3=4k_het/Sω=4k_het/S√(8RT/π M)
 (2) where S is the surface-to-volume ratio of aerosols (m −1 ) and is measured using these instruments for particle size distribution, ω is the mean velocity of NH 3 molecules, R is the ideal gas constant, T is the air temperature (K), and M is the molecular weight of NH 3 (kg mol −1 ). The uncertainty for calculating the γ NH3 is discussed in the SI (Supplementary Figs. 19 and 20 and Supplementary Table 2 ). The aerosol water content (AWC) and pH were estimated by combining an aerosol thermodynamic model and the measured particle composition with T and RH, assuming that the aerosol system was in equilibrium. The ISORROPIA II model, which is widely used in aerosol pH estimation [48] , [49] , [53] , [102] , was used in the “forward” mode assuming that the particles were in the “metastable” phase state to predict the concentration of H + per volume of air ( c H+ , μg m −3 ) and the concentration of AWC (μg m −3 ) [46] , [54] . The pH is then calculated according to 
    pH=-log _101000γ_H^+c_H^+/AWC
 (3) where γ H+ is the activity coefficient of H + (assumed to be 1.0) [46] , [54] . Under such an assumption, the calculated pH is pH F indeed based on only the free-H + molality [80] . Both the inorganic species and part of the organic species in particles are hygroscopic. Similar to previous work [48] , [49] , [53] , [102] , aerosol pH and AWC were predicted with only inorganic species because pH prediction was not highly sensitive to water uptake by organic species [53] , and the mass fraction of organic matter-induced particle water accounted for only 5% of the total AWC in Beijing [103] . AWC becomes very small when RH is low, subsequently introducing considerable uncertainty to aerosol pH [47] , [53] , [80] . Thus, we only calculated the aerosol pH for data with RH higher than 35% [80] . Identification of factors affecting aerosol pH A random forest model (RF) was used to identify the crucial factors that affect aerosol pH. We used the classification and regression tree (CART) decision tree as the base learner for integrated learning. According to the bagging algorithm [65] , several independent and identically distributed training subsets are randomly obtained from the training set, and numerous decision trees are constructed according to the training subsets. We used the Gini coefficients as the criteria for node feature selection. Supplementary Fig. 21 shows the error loss during the training of the model. It can be seen that no underfitting or overfitting occurred in this model. In addition, the aerosol pH predicted by the RF model has a satisfactory correlation coefficient ( R = 0.95) with that calculated using the ISORRPIA-II model. The relative standard deviation (RSD) is 4.61%. Source apportionment of PM 2.5 in Shijiazhuang was performed using a receptor model (positive matrix factor, PMF, EPA 5.0). The model was fed with the hourly mean concentrations ( c ij ) and the uncertainties ( S ij ) of species, including water-soluble ions, OC, EC, and heavy metals. The S ij for each species was calculated using measurement uncertainties (MU%) and method detection limits (MDL) [104] . If c ij ≤ MDL, 
    S_ij=5/6×MDL
 (4) Unless 
    S_ij=√((MU×c_ij)^2+(0.5MDL)^2)
 (5) The dataset from May 13, 2019, to November 15, 2020, was used for source apportionment because of the availability of the heavy metal analyzer.